Auto-regulatory RNA editing fine-tunes mRNA re-coding and complex behaviour inDrosophila Auto-regulatory feedback loops are a common molecular strategy used to optimize protein function. In Drosophila , many messenger RNAs involved in neuro-transmission are re-coded at the RNA level by the RNA-editing enzyme, dADAR, leading to the incorporation of amino acids that are not directly encoded by the genome. dADAR also re-codes its own transcript, but the consequences of this auto-regulation in vivo are unclear. Here we show that hard-wiring or abolishing endogenous dADAR auto-regulation dramatically remodels the landscape of re-coding events in a site-specific manner. These molecular phenotypes correlate with altered localization of dADAR within the nuclear compartment. Furthermore, auto-editing exhibits sexually dimorphic patterns of spatial regulation and can be modified by abiotic environmental factors. Finally, we demonstrate that modifying dAdar auto-editing affects adaptive complex behaviours. Our results reveal the in vivo relevance of auto-regulatory control over post-transcriptional mRNA re-coding events in fine-tuning brain function and organismal behaviour. ADARs (adenosine deaminases that act on RNA) mediate RNA editing through the deamination of adenosine (A) to inosine (I) in double-stranded RNA (dsRNA) templates [1] . Intriguingly, in mammals and insects, messenger RNAs that encode proteins involved in electrical and chemical neuro-transmission are highly over-represented in the population of transcripts known to undergo editing [2] , [3] . Importantly, as inosine is interpreted as guanosine by the ribosome, RNA editing in exonic regions often leads to amino-acid re-coding, and thus translation into proteins that are not literally encoded by genomic DNA templates [4] . Analysis of mutations in adar alleles in several diverse model organisms has demonstrated that RNA editing is crucial to neuronal function and integrity across a broad range of phyla [5] , [6] , [7] . Loss of mouse ADAR2 expression leads to early mortality associated with severe seizures [5] . Null mutations in the single Drosophila adar ( dAdar ), while not lethal, result in extreme adult-stage behavioural defects, including un-coordinated locomotion, temperature-sensitive paralysis, seizures, and a lack of the male courtship display [6] . In the majority of dADAR target mRNAs, between one and several adenosines are deaminated, often at low-to-moderate levels [2] , [8] , and studies have thus far demonstrated relatively subtle modifications of ion-channel function through dADAR-mediated amino-acid re-coding [9] , [10] , suggesting that RNA editing generally acts to 'fine-tune' protein activity [11] . The extreme phenotype observed in dAdar null flies may therefore reflect the cumulative action of dADAR's functional pleiotropy. Comparative genomics approaches and serendipitous observations have identified a host of edited adenosines in mRNAs encoding ion channels and regulators of exo- and endo-cytosis [2] , [12] , [13] , [14] , [15] . Similarly, mammalian ADAR substrates include several G-protein-coupled receptors and ion channels [16] . Recent bioinformatic analysis and deep sequencing experiments have identified hundreds of additional potential ADAR targets in both the Drosophila and human transcriptomes [17] , [18] , [19] . Interestingly, hyper-activity of ADARs has also been shown to cause physiological and behavioural abnormalities. Overexpression of ADAR2 in mice leads to both adult-onset obesity and increased anxiety-related behaviours [20] , [21] , whereas global overexpression of a dADAR isoform in Drosophila results in larval lethality [22] . These observations imply that precise control of mRNA re-coding is essential for development and adaptive behaviour. Intriguingly, both mammalian and Drosophila ADARs have evolved distinct auto-regulatory feedback loops as a mechanism to alter enzymatic activity through deamination of adenosines within their own transcripts [23] , [24] . Rodent ADAR2 auto-editing acts as a negative feedback mechanism by generating a novel splicing acceptor site (AA→AI), leading to an amino-terminal frame-shift and translation of a truncated ADAR2 isoform at reduced levels [24] . Correspondingly, abolition of ADAR2 auto-editing in vivo increases ADAR2 expression and editing at several target adenosines [25] . In contrast, dAdar auto-editing results in a serine to glycine (S→G) coding change in the carboxy-terminal catalytic domain [23] . Auto-editing of dAdar mRNA is developmentally regulated, occurring predominantly at the pupal and adult stages, and is mediated by a complementary sequence within the edited exon [22] , [23] . In vitro experiments using two dADAR substrates, supported by in vivo data gained from expression of differentially edited dADAR transgenes, indicate that auto-editing acts to reduce dADAR activity, suggesting an evolutionary convergence in function of dADAR and ADAR2 auto-regulation [22] . However, it is unknown whether dAdar auto-editing acts globally to reduce editing at all target adenosines in vivo or, rather, to modify particular target adenosines in a substrate-specific manner. To understand how dAdar auto-regulation shapes RNA-editing patterns in vivo , we genetically engineered Drosophila with either fully edited or un-edited dAdar alleles, and assessed editing levels across 100 adenosines in various dADAR mRNA targets in multiple male and female tissues, revealing a non-uniform modification of complex spatially regulated patterns of mRNA re-coding. Furthermore, we show that both preventing and constitutive hard-wiring of dAdar auto-regulation adversely affects adult-stage behaviours. Our results shed light on the adaptive importance of fine-tuning the 'fine-tuner' in Drosophila . Modifying the edited residue in the dAdar locus The auto-edited serine residue of dADAR is conserved throughout metazoan dADAR and ADAR2 homologues and structurally maps to a loop near the active site in the human ADAR2 crystal structure [26] ( Fig. 1a,b ). To determine the in vivo significance of auto-editing, we performed ends-out homologous recombination [27] on the endogenous X-linked dAdar locus to generate Drosophila with either constitutive serine (S) or glycine (G) residues ( Fig. 1c ). An allele producing only auto-edited dADAR protein ( dAdar G ) was engineered by mutating the edited adenosine of the serine codon ( A GT) to guanosine ( G GT), converting it to an obligate glycine codon. Conversely, a dAdar S allele, producing only un-edited dADAR, was generated by altering the same serine codon to its degenerate counterpart (TCT), rendering A-to-I modification impossible. A dAdar allele containing a single intronic loxP site but with no alteration at the edited serine residue ( dAdar WTLoxP ) served as a wild-type control. In addition, we generated identical targeted recombinant flies with the above alleles and also containing an HA-epitope tag at the 3′ terminus of the dAdar -coding sequence ( Fig. 1c ). We have previously shown that the HA-tag has no effect on dADAR activity on several known targets [28] , and western blot analyses revealed that modifying auto-editing has no significant effect on levels of dADAR protein expression ( Fig. 1d ). We therefore used the above lines to investigate the functional consequences of auto-editing in a genetic background, where the remaining endogenous control of dADAR expression is intact. 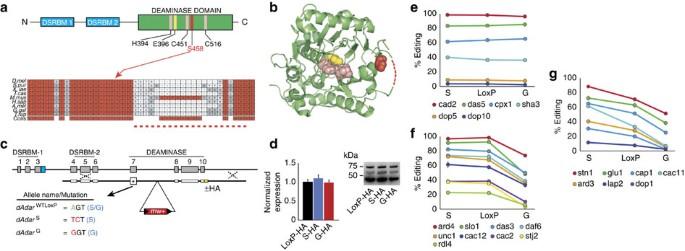Figure 1:dAdarauto-editing selectively modulates mRNA re-coding. (a) The auto-edited residue resides within the C-terminal catalytic deaminase domain, which is downstream of the two double-strand RNA-binding motifs (DSRBMs). Zinc-ion coordinating residues (H394, C541 and C516) are shown in pink, and the proton-shuttling residue (E396) is shown in yellow. Auto-editing results in an amino-acid substitution (S458G), at a residue highly conserved in ADAR2 homologues. (b) The orthologous position in the human ADAR2 crystal structure (PDB-1ZY7) is close to the active site of the deaminase domain26. Dotted lines indicate unstructured region. (c) Schematic of thedAdarlocus and nomenclature for the three engineereddAdaralleles. (d) ModifyingdAdarauto-editing does not affect dADAR expression (n=5–6 western blots from 3 separate head-protein samples;P>0.63, one-way ANOVA with Tukey's HSDpost-hoctest). Values are presented as dADAR (top band)/actin (lower band). Middle band: nonspecific signal. (e–g) Examples of edited adenosines that show no alteration (e), a mono- (f) or bi-directional (g) shift in editing levels indAdarSanddAdarGmale heads when compared withdAdarWTLoxP. Mean values for each site were defined as significantly different (P<0.05) fromdAdarWTLoxPusing one-way ANOVA with Dunnettpost-hoctest (n=3–14 PCRs per site). Error bars, s.e.m. Figure 1: dAdar auto-editing selectively modulates mRNA re-coding. ( a ) The auto-edited residue resides within the C-terminal catalytic deaminase domain, which is downstream of the two double-strand RNA-binding motifs (DSRBMs). Zinc-ion coordinating residues (H394, C541 and C516) are shown in pink, and the proton-shuttling residue (E396) is shown in yellow. Auto-editing results in an amino-acid substitution (S458G), at a residue highly conserved in ADAR2 homologues. ( b ) The orthologous position in the human ADAR2 crystal structure (PDB-1ZY7) is close to the active site of the deaminase domain [26] . Dotted lines indicate unstructured region. ( c ) Schematic of the dAdar locus and nomenclature for the three engineered dAdar alleles. ( d ) Modifying dAdar auto-editing does not affect dADAR expression ( n =5–6 western blots from 3 separate head-protein samples; P >0.63, one-way ANOVA with Tukey's HSD post-hoc test). Values are presented as dADAR (top band)/actin (lower band). Middle band: nonspecific signal. ( e–g ) Examples of edited adenosines that show no alteration ( e ), a mono- ( f ) or bi-directional ( g ) shift in editing levels in dAdar S and dAdar G male heads when compared with dAdar WTLoxP . Mean values for each site were defined as significantly different ( P <0.05) from dAdar WTLoxP using one-way ANOVA with Dunnett post-hoc test ( n =3–14 PCRs per site). Error bars, s.e.m. Full size image dAdar editing reduces RNA editing at certain target mRNAs A-to-I signatures have been detected in a wide range of mRNAs encoding ion channels and regulators of endo- and exo-cytosis [2] . To comprehensively determine the influence of dAdar auto-editing on mRNA re-coding, we examined editing levels at 100 adenosines in 23 mRNAs amplified from dAdar WTLoxP , dAdar S and dAdar G male head complementary DNA ( Figs 1e–g and 2a ; Supplementary Fig. S1 ; Supplementary Table S1 ; Supplementary Data 1 , 2 , 3 , 4 , 5 , 6 ). Although recent deep sequencing data has suggested the existence of potentially hundreds of previously unidentified editing targets [29] , we limited our analysis to neuronally expressed mRNAs in which mixed A/G peaks have been shown to be abolished in a dAdar null background, and whose orthologous mRNAs exhibit signatures of editing in other Drosophilid species. The 100 adenosines analysed represent >80% of the ~120 known editing sites that fit the above criteria. We were able to delineate three categories of editing sites from our initial dataset: adenosines that were completely insensitive to the edited state of dADAR ( Fig. 1e ); adenosines where elimination of auto-editing was inconsequential, yet exhibited a significant reduction in editing level on hard-wiring of dAdar auto-editing ( Fig. 1f ); and finally, adenosines which exhibited a bi-directional response to elimination or hard-wiring of auto-editing ( Fig. 1g ). Examples of each class could even be found in the same mRNA ( Supplementary Fig. S2a,b ). Thus, it is unlikely that the responsiveness of a given site to dADAR's auto-regulatory state is due to transcript abundance. Importantly, the above classes were not biased towards adenosines with particular levels of editing, and comprise diverse mRNAs ( Supplementary Fig. S2c,d ). Thus, dAdar auto-editing acts as a negative auto-regulatory feedback mechanism to selectively modulate dADAR activity on particular target adenosines in the male Drosophila head. 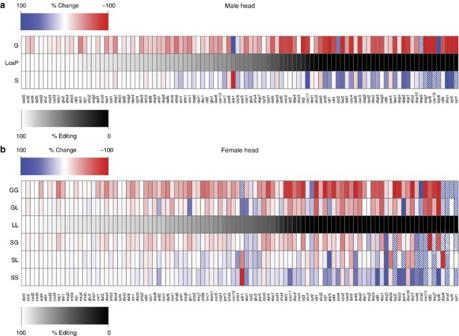Figure 2: Inhibiting or hard-wiringdAdarauto-regulation results in widespread alterations in RNA editing of target adenosines. (a) Heat-map representation of alterations in editing at 100 adenosines indAdarSanddAdarGmales relative todAdarWTLoxPcontrols. All PCRs were performed using male head cDNA. Data are derived fromn≥3 RT–PCRs for each adenosine, and are presented in rank order relative to the endogenous editing levels indAdarWTLoxP. Dashed boxes indicate a >100% increase. (b) Heat map showing levels of editing at 100 adenosines in mRNAs amplified fromdAdarS/S,dAdarS/L,dAdarS/G,dAdarL/L,dAdarG/LanddAdarG/Gfemale heads, presented in rank order relative to the endogenous editing levels indAdarL/L. L indicates thedAdarWTLoxPallele. Figure 2: Inhibiting or hard-wiring dAdar auto-regulation results in widespread alterations in RNA editing of target adenosines. ( a ) Heat-map representation of alterations in editing at 100 adenosines in dAdar S and dAdar G males relative to dAdar WTLoxP controls. All PCRs were performed using male head cDNA. Data are derived from n ≥3 RT–PCRs for each adenosine, and are presented in rank order relative to the endogenous editing levels in dAdar WTLoxP . Dashed boxes indicate a >100% increase. ( b ) Heat map showing levels of editing at 100 adenosines in mRNAs amplified from dAdar S/S , dAdar S/L , dAdar S/G , dAdar L/L , dAdar G/L and dAdar G/G female heads, presented in rank order relative to the endogenous editing levels in dAdar L/L . L indicates the dAdar WTLoxP allele. Full size image To test whether the selective negative-feedback effect of dAdar auto-editing observed in male heads was tissue- and/or sex-specific, we analysed the same set of 100 adenosines using RNA derived from male antennal, eye and thorax cDNA ( Supplementary Data 1 , 2 , 3 ), and head and thorax cDNA from all possible female allelic combinations ( Fig. 2b ; Supplementary Data 1 , 2 , 3 , 4 , 5 , 6 ), and found a similar reduction in editing levels across many dADAR targets in all dAdar G hemi- and homo-zygotic tissues. Furthermore, in both male and female head and thorax tissues, inhibiting the intrinsic regulation of dAdar auto-editing resulted in global alterations in the relative quantitative dynamics of RNA editing of the 100 adenosines studied ( Fig. 3a–d ). 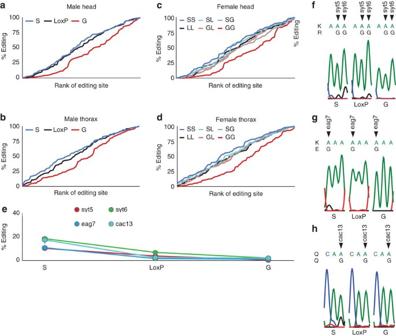Figure 3: Hard-wiring ofdAdarauto-editing modifies the quantitative pattern of RNA editing. (a,b) Rank-ordered editing levels at 100 adenosines amplified fromdAdarS,dAdarWTLoxPanddAdarGmale head (a) and thorax tissues (b). Each population is rank-ordered independently to assess the relative abundance of adenosines edited at low, medium and high levels. Note the substantial downward shift in the rank ordering of editing sites amplified fromdAdarGtissues compared with bothdAdarWTLoxPanddAdarS. (c,d) Rank-ordered editing levels at 100 adenosines amplified from head (c) and thorax (d) tissue of the six female allelicdAdarcombinations. Note the substantial downward shift in the rank ordering of editing sites amplified fromdAdarG/Gtissues compared with all other allelic combinations. (e–h) Editing levels at novel editing sites that were solely or predominantly detected indAdarShemi- and homo-zygotic backgrounds. All of the novel sites were detected at relatively low levels (e). Editing atSynaptotagmin-1site 5 (syt5) (f) andeagsite 7 (eag7) (g) lead to the amino-acid substitutions K→R and K→E, respectively. RNA editing atsynaptotagmin-1site 6 (syt6) (f) andcacophonysite 13 (cac13) (h) result in synonymous changes. Data are derived fromn≥3 RT–PCRs for each adenosine. Error bars, s.e.m. Figure 3: Hard-wiring of dAdar auto-editing modifies the quantitative pattern of RNA editing. ( a,b ) Rank-ordered editing levels at 100 adenosines amplified from dAdar S , dAdar WTLoxP and dAdar G male head ( a ) and thorax tissues ( b ). Each population is rank-ordered independently to assess the relative abundance of adenosines edited at low, medium and high levels. Note the substantial downward shift in the rank ordering of editing sites amplified from dAdar G tissues compared with both dAdar WTLoxP and dAdar S . ( c , d ) Rank-ordered editing levels at 100 adenosines amplified from head ( c ) and thorax ( d ) tissue of the six female allelic dAdar combinations. Note the substantial downward shift in the rank ordering of editing sites amplified from dAdar G/G tissues compared with all other allelic combinations. ( e–h ) Editing levels at novel editing sites that were solely or predominantly detected in dAdar S hemi- and homo-zygotic backgrounds. All of the novel sites were detected at relatively low levels ( e ). Editing at Synaptotagmin-1 site 5 (syt5) ( f ) and eag site 7 (eag7) ( g ) lead to the amino-acid substitutions K→R and K→E, respectively. RNA editing at synaptotagmin-1 site 6 (syt6) ( f ) and cacophony site 13 (cac13) ( h ) result in synonymous changes. Data are derived from n ≥3 RT–PCRs for each adenosine. Error bars, s.e.m. Full size image In addition, we observed novel editing sites that were only apparent in bulk RT–PCR from dAdar S backgrounds ( Fig. 3e–h ). One of these, a K→E substitution in the cyclic nucleotide-binding domain of eag , is 100 nucleotides from the closest known editing site [2] , suggesting the presence of a novel dADAR substrate that is only deaminated in neurons where dAdar auto-editing is very low or absent. This data raises the possibility of the existence of an undefined number of adenosines where editing occurs only when high levels of the dADAR S isoform are present. Spatial control of dAdar editing Previous in vitro experiments have suggested that dAdar mRNA is efficiently deaminated by unedited dADAR protein, but the edited version is far less effective [22] . This observation provided a clear prediction that the presence of either of our modified dAdar alleles should shift the auto-editing of a wild-type allelic counterpart in the opposite direction, that is, total auto-editing levels in dAdar WTLoxP / dAdar S and dAdar WTLoxP / dAdar G heterozygotes should tend towards a similar equilibrium value, presumably close to wild-type levels (~50%; Fig. 4a ). In contrast, however, we found a linear increase in auto-editing levels when comparing dAdar WTLoxP / dAdar S dAdar WTLoxP / dAdar WTLoxP and dAdar WTLoxP / dAdar G female heads ( Fig. 4a ), indicating that auto-editing of dAdar mRNA is insensitive to the edited status of co-expressed dADAR proteins, and that there is no compensation at the level of auto-editing. 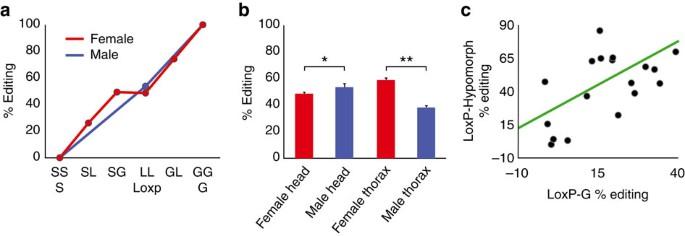Figure 4: Spatial regulation of dADAR auto-editing. (a) Total auto-editing levels at a wild-typedAdarlocus in combination with engineered mutations indAdarauto-editing.dAdarShemi- and homo-zygotes are defined as having 0% auto-editing, whereasdAdarGis 100%. Auto-editing levels in the remaining allelic combinations were determined experimentally (Methods). L, wild-type LoxP allele. (b) Auto-editing levels indAdarWTLoxPmale and female head and thoracic tissues.n=5–8 PCRs. *:P<0.05, **:P<0.005, Mann–WhitneyU-test. (c) Correlation between the reduction in editing at 18 adenosines indAdarGanddAdarhypmale heads. Error bars, s.e.m. Figure 4: Spatial regulation of dADAR auto-editing. ( a ) Total auto-editing levels at a wild-type dAdar locus in combination with engineered mutations in dAdar auto-editing. dAdar S hemi- and homo-zygotes are defined as having 0% auto-editing, whereas dAdar G is 100%. Auto-editing levels in the remaining allelic combinations were determined experimentally (Methods). L, wild-type LoxP allele. ( b ) Auto-editing levels in dAdar WTLoxP male and female head and thoracic tissues. n =5–8 PCRs. *: P <0.05, **: P <0.005, Mann–Whitney U -test. ( c ) Correlation between the reduction in editing at 18 adenosines in dAdar G and dAdar hyp male heads. Error bars, s.e.m. Full size image Furthermore, we observed strong sexual dimorphism of auto-editing levels in the thorax, but only a small difference between male and female heads ( Fig. 4b ), illustrating that dAdar auto-regulation can be spatially controlled in a sex-specific manner. To test whether this spatial variation was conserved amongst other Drosophilids , we examined auto-editing in four other members of the D. melanogaster subgroup: D. simulans , D. sechellia , D. yakuba and D. erecta ( Fig. 5a ). We found that robust sexual dimorphism in thoracic auto-editing was conserved in D. simulans and D. sechellia , the closest species to D. melanogaster , whereas in the more divergent species D. yakuba and D. erecta , only subtle differences were observed ( Fig. 5b ). Furthermore, each species within the D. melanogaster subgroup possessed a distinct level of auto-editing in male and female head and thorax tissue ( Fig. 5c-f ), indicating that spatial control over dADAR auto-editing is fine-tuned in a species-specific manner, potentially resulting in distinct landscapes of RNA-editing levels of target transcripts across even recently diverged Drosophilid species. 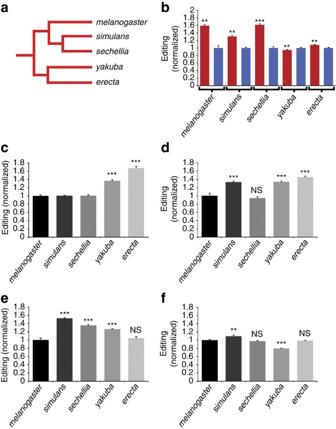Figure 5: dADAR auto-editing inDrosophilidspecies of theD. melanogastersubgroup. (a) Schematic phylogenetic tree indicating evolutionary relationships between each species within theD. melanogastersubgroup. (b) dADAR auto-editing in male (blue) and female (red) thoraxes in the five species of theD. melanogastersubgroup. Values are normalized to the mean auto-editing level in male thoraxes for each species. **:P<0.005, ***:P<0.0005, Mann–WhitneyU-test;n=5–8 PCRs per tissue. (c–f) dADAR auto-editing levels in male heads (c), male thoraxes (d), female heads (e) and female thoraxes (f) in the five species of theD. melanogastersubgroup. dADAR auto-editing levels inD. sechellia,D. simulans,D. yakubaandD. erectawere normalized toD. melanogasterauto-editing levels for each tissue-type. **:P<0.005, ***:P<0.0005, NS:P>0.05, one-way ANOVA with Dunnettpost-hoctest;n=5–8 PCRs per tissue. Error bars, s.e.m. Figure 5: dADAR auto-editing in Drosophilid species of the D. melanogaster subgroup. ( a ) Schematic phylogenetic tree indicating evolutionary relationships between each species within the D. melanogaster subgroup. ( b ) dADAR auto-editing in male (blue) and female (red) thoraxes in the five species of the D. melanogaster subgroup. Values are normalized to the mean auto-editing level in male thoraxes for each species. **: P <0.005, ***: P <0.0005, Mann–Whitney U -test; n =5–8 PCRs per tissue. ( c–f ) dADAR auto-editing levels in male heads ( c ), male thoraxes ( d ), female heads ( e ) and female thoraxes ( f ) in the five species of the D. melanogaster subgroup. dADAR auto-editing levels in D. sechellia , D. simulans , D. yakuba and D. erecta were normalized to D. melanogaster auto-editing levels for each tissue-type. **: P <0.005, ***: P <0.0005, NS: P >0.05, one-way ANOVA with Dunnett post-hoc test; n =5–8 PCRs per tissue. Error bars, s.e.m. Full size image dAdar editing alters its nuclear localization What is the mechanism by which auto-editing selectively reduces dADAR function? We recently engineered a novel hypomorphic allele of dAdar ( dAdar hyp ), in which dADAR expression is reduced by ~80% (ref. 28 ). In this background, editing at many sites, but not all, is significantly reduced. Similarly to dAdar hyp animals, males and females hemi- or homo-zygous for the dAdar G allele also show reduced editing at a subset of adenosines ( Fig. 2 ). Interestingly, for the editing sites that showed a significant reduction in dAdar G males, we found a significant correlation between the degree of reduction in both dAdar G and dAdar hyp heads ( r =0.57, P =0.008, permutation test; Fig. 4c ). Thus, in essence, auto-editing seems to post-transcriptionally phenocopy a known hypomorphic allele of dAdar . To explore this further, we examined the localization of dADAR, in our various genetic backgrounds, using HA-tagged versions of each allele ( Fig. 1a ), with the underlying hypothesis that auto-editing might in some way be lowering the effective concentration of dADAR within the nuclear compartment. Mammalian ADARs have been shown to localize to the nucleolus and alter their localization in response to substrate abundance [30] . dADAR transgenes comparable to the dAdar WTLoxP , and dAdar S alleles also localized to the nucleolus when ectopically expressed in third instar larval salivary gland nuclei ( Supplementary Fig. S3a ). We next examined the endogenous localization of dADAR isoforms in neuronal nuclei of the adult brain. Both ectopically expressed dADAR transgenes and endogenous dADAR protein, derived from all HA-tagged dAdar alleles, localized to within the nuclear envelope ( Supplementary Fig. S3b,c ). Within the nucleus, we observed two patterns of expression that were common to all engineered dADAR isoforms ( Fig. 6a–c ). Firstly, concordant with the localization of dADAR expressed from transgenes in larval salivary glands, we observed a strong co-localization with the nucleolar marker fibrillarin. dADAR levels in all genetic backgrounds studied were often strongly elevated in the nucleolus relative to the expression in the remainder of the nucleus. Secondly, diffuse expression was detected throughout the non-nucleolar region of the nucleus. However, we also observed an intriguing mode of localization that was robustly observed in neurons expressing the dADAR G-HA isoform, but not the dADAR S-HA isoform, characterized by the presence of intense punctae of nuclear dADAR expression outside the nucleolus, smaller in size relative to the nucleolus, and distinct from the general diffuse staining observed within the nucleus (shown in Fig. 6d ; see also Fig. 6a–c and Supplementary Fig. S3c ). 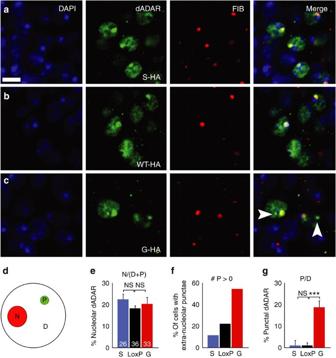Figure 6: Auto-editing modifies the sub-nuclear localization of dADAR. (a–c) Confocal slices illustrating the nuclear localization of HA-tagged dADARS(a), dADARWTLoxP(b) and dADARG(c) alleles in the adult male nervous system. To control for spatial differences in dADAR localization, slices were obtained from nuclei surrounding the antennal lobes. All dADAR alleles co-localized with DAPI-stained DNA (blue) and the nucleolus (stained with fibrillarin, red). (d) Schematic diagram illustrating quantification of the regional dADAR signal intensity in the nucleolus (N) compared with dispersed (D) or punctate (P, arrowheads) extra-nucleolar staining between WTLoxP-HA, S-HA and G-HA dADARs. (e) Altering auto-editing does not alter the proportion of total dADAR signal co-localizing with fibrillarin. (f) Proportion of neurons exhibiting ≥0 extra-nucleolar puncta in the three experimental genotypes. Number of cells used for computational analysis: dADARWTloxP−HA—36; dADARS-HA—26; dADARG−HA—33. (g) Proportion of dADAR signal that is both non-nucleolar and punctate in the three experimental genotypes. ***:P<0.0005, one-way ANOVA with Dunnettpost-hoctest. Error bars, s.e.m. Images were derived fromn≥5 brains for each genotype. Scale bars, 5 μm. Figure 6: Auto-editing modifies the sub-nuclear localization of dADAR. ( a–c ) Confocal slices illustrating the nuclear localization of HA-tagged dADAR S ( a ), dADAR WTLoxP ( b ) and dADAR G ( c ) alleles in the adult male nervous system. To control for spatial differences in dADAR localization, slices were obtained from nuclei surrounding the antennal lobes. All dADAR alleles co-localized with DAPI-stained DNA (blue) and the nucleolus (stained with fibrillarin, red). ( d ) Schematic diagram illustrating quantification of the regional dADAR signal intensity in the nucleolus (N) compared with dispersed (D) or punctate (P, arrowheads) extra-nucleolar staining between WTLoxP-HA, S-HA and G-HA dADARs. ( e ) Altering auto-editing does not alter the proportion of total dADAR signal co-localizing with fibrillarin. ( f ) Proportion of neurons exhibiting ≥0 extra-nucleolar puncta in the three experimental genotypes. Number of cells used for computational analysis: dADAR WTloxP−HA —36; dADAR S-HA —26; dADAR G−HA —33. ( g ) Proportion of dADAR signal that is both non-nucleolar and punctate in the three experimental genotypes. ***: P <0.0005, one-way ANOVA with Dunnett post-hoc test. Error bars, s.e.m. Images were derived from n ≥5 brains for each genotype. Scale bars, 5 μm. Full size image We computationally analysed the relative co-localization of dADAR with the nucleolus and the abundance of extra-nucleolar punctae in the HA-tagged dADAR backgrounds ( Supplementary Fig. S4 ). All endogenous HA-tagged dADARs co-localized with the nucleolus to a degree that was independent of auto-editing status ( Fig. 6e ). In contrast, the number of nuclei exhibiting extra-nucleolar punctae, and the intensity of the dADAR signal within such punctae, exhibited striking variation depending on the auto-edited status of dADAR ( Fig. 6f,g ; Supplementary Fig. S5 ). In dADAR S-HA neurons, dADAR-positive extra-nucleolar punctae were detected in only ~10% of nuclei, whereas this value rose to >50% in dADAR G-HA neurons ( Fig. 6f ). Furthermore, the intensity of the dADAR signal in extra-nucleolar punctae was significantly higher in dADAR G-HA neurons relative to either unedited or wild-type HA-tagged dADARs ( Fig. 6g ). We observed a similar pattern of localization using a different anti-HA antibody ( Supplementary Fig. S6 ), indicating that this effect is not antibody-specific. These results suggest that auto-editing leads to the sequestration of dADAR G isoform to a distinct nuclear compartment, perhaps reflecting binding to a form of dsRNA that is not bound by dADAR S-HA stably enough to be detectable by confocal microscopy. We hypothesize that this localized depot of dADAR G effectively lowers the concentration of total dADAR at active sites of target transcription, generating a molecular phenocopy of a dAdar hypomorph to which only specific dADAR targets are sensitive. dAdar editing modulates adult behaviour A common theme of ADAR mutations in several higher metazoan model genetic systems is the disruption of normal nervous system function [5] , [6] , [7] , [28] . We therefore asked whether the relatively subtle changes in editing observed in the dAdar S and dAdar G backgrounds could also confer abnormal adult-stage behaviours. We assessed adult locomotor patterns using both automated horizontal single-fly and vertical population monitors. In constant dark conditions, all genotypes exhibited rhythmic locomotor patterns ( Supplementary Fig. S7 ), indicating that the circadian clock is intact in the recombinant lines. However, in 12-h light: 12-h dark conditions, we observed a reduction in morning anticipation in dAdar G compared with dAdar WTLoxP and dAdar S males ( Fig. 7a,b ). The anticipation of morning is an output of a subset of the circadian neuronal network, and interestingly is also absent in dAdar hypomorphs [28] , [31] . To quantify the degree of increase in locomotor activity in the hours preceding the onset of morning, we calculated the total number of beam breaks occurring in the 3 hours before lights-on divided by the total in the 6 hours before lights-on (that is, a value of 0.5 indicates no anticipation). Although dAdar G males did show a detectable degree of anticipation (0.72±0.02), the level was significantly reduced relative to both dAdar WTLoxP (0.82±0.02; P =0.0059, ANOVA with Dunnett post-hoc test) and dAdar S (0.81±0.02; P =0.022) males. In both single-fly and population settings ( Fig. 7c,d ), altering auto-editing did not change locomotor activity relative to dAdar WTLoxP , although dAdar S males were significantly more active than dAdar G under horizontal conditions ( Fig. 7c ). In addition, in the vertical assay, the proportion of time dAdar S males spent towards the top of the vial was significantly lower compared with dAdar WTLoxP and dAdar G males, suggesting that loss of auto-editing impairs normal climbing ability while sparing general horizontal locomotor activity ( Fig. 7e ). 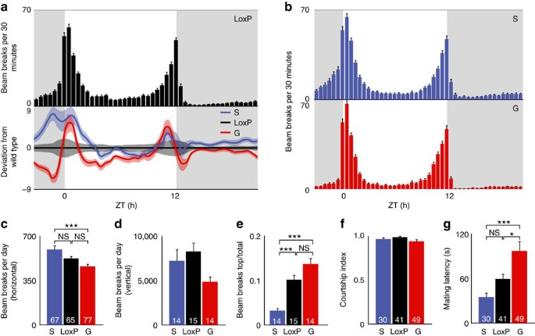Figure 7: Dysregulation ofdAdarauto-editing alters complex behaviours. (a) Locomotor profile ofdAdarWTLoxPcontrol males under 12-h light: 12-h dark (LD) conditions. Top panel, bar graph showing mean LD activity indAdarWTLoxPmales (n=65). Grey background indicates lights-off; white background indicates lights-on. Lower panel, mean locomotion indAdarS(n=67) anddAdarG(n=77) males, normalized todAdarWTLoxP. Light bars indicate s.e.m. (b) Locomotor profiles ofdAdarSanddAdarGmales. (c) Total locomotor levels derived from single-fly activity data. (d–e) Total locomotor levels (d) and relative climbing ability (e) derived from vertical population activity monitors. Climbing was quantified by normalizing the beams breaks in the top third of the vertical vial to the total number of beam breaks.dAdarWTLoxP:n=15 vials each containing 5 male flies;dAdarS:n=14;dAdarG:n=14. (f–g) Courtship indAdarWTLoxP,dAdarSanddAdarGmales. Although the fraction of time spent courting females was not significantly different between experimental and control genotypes (f),dAdarGmales (n=49) took significantly longer to initiate courtship relative todAdarWTLoxP(n=41) ordAdarS(n=30) males (g). *:P<0.05, ***:P<0.0005, one-way ANOVA with Tukey's HSDpost-hoctest. Error bars, s.e.m. Figure 7: Dysregulation of dAdar auto-editing alters complex behaviours. ( a ) Locomotor profile of dAdar WTLoxP control males under 12-h light: 12-h dark (LD) conditions. Top panel, bar graph showing mean LD activity in dAdar WTLoxP males ( n =65). Grey background indicates lights-off; white background indicates lights-on. Lower panel, mean locomotion in dAdar S ( n =67) and dAdar G ( n =77) males, normalized to dAdar WTLoxP . Light bars indicate s.e.m. ( b ) Locomotor profiles of dAdar S and dAdar G males. ( c ) Total locomotor levels derived from single-fly activity data. ( d–e ) Total locomotor levels ( d ) and relative climbing ability ( e ) derived from vertical population activity monitors. Climbing was quantified by normalizing the beams breaks in the top third of the vertical vial to the total number of beam breaks. dAdar WTLoxP : n =15 vials each containing 5 male flies; dAdar S : n =14; dAdar G : n =14. ( f–g ) Courtship in dAdar WTLoxP , dAdar S and dAdar G males. Although the fraction of time spent courting females was not significantly different between experimental and control genotypes ( f ), dAdar G males ( n =49) took significantly longer to initiate courtship relative to dAdar WTLoxP ( n =41) or dAdar S ( n =30) males ( g ). *: P <0.05, ***: P <0.0005, one-way ANOVA with Tukey's HSD post-hoc test. Error bars, s.e.m. Full size image Because both null and hypomorphic mutations in dAdar result in abnormal mating behaviours [6] , [28] , we also investigated courtship in recombinant males with hard-wired or abolished dADAR auto-editing. Whereas the total time spent courting females was equivalent to wild-type, dAdar G males initiated courtship significantly slower than dAdar WTLoxP controls or dAdar S males ( Fig. 7f,g ). Thus, homeostatic control of dADAR function through auto-regulation modulates behaviours that are subject to natural selection and would be expected to affect fitness. Abiotic modulation of dAdar editing dADAR auto-regulation is subject to both temporal [23] and spatial control ( Figs 4b and 5b ). We were interested in examining whether external abiotic factors were also able to modulate dADAR auto-editing. To do so, we raised wild-type Drosophila at 25 °C and then exposed newly eclosed males to one of three test temperatures for 72 h: 15, 25 or 35 °C. We subsequently examined the magnitude of editing in the dAdar transcript. Interestingly, we observed a bi-directional alteration in the levels of dADAR auto-editing: lowering the ambient temperature by 10 °C resulted in a 20% increase in auto-editing. In contrast, an increase of 10 °C led to a 30% reduction in auto-editing levels ( Fig. 8a,b ). These results point to an intriguing interaction between changing environmental conditions and post-transcriptional mRNA re-coding events that possess the capacity to modulate adult-stage behaviours. 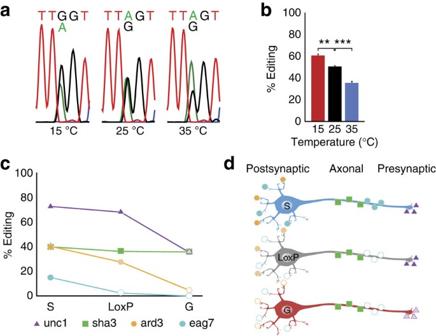Figure 8: Environmental modulation of dADAR auto-editing. (a–b) Auto-editing levels in adult males kept at differing temperatures for 72 h. Representative electropherograms are shown in (a), and averaged data in (b). Experimental temperatures are indicated.n=3 RT–PCRs per population. **:P<0.005, ***:P<0.0005, one-way ANOVA with Dunnettpost-hoctest. Error bars, s.e.m. (c) Model depicting the functional consequences of neuron-to-neuron variation in auto-editing. The graph depicts the change in editing of four substrate adenosines in thedAdarWTLoxP,dAdarS, anddAdarGgenetic backgrounds.Shakersite 3 (sha3) belongs to the category of editing sites that was insensitive to the edited status ofdAdar.Unc-13site 1 (unc1) belongs to the class of editing sites that displayed no effect on elimination of auto-editing, but exhibited a significant reduction on hard-wiring ofdAdarauto-editing, whereasardsite 3 (ard3) belongs to the group of editing sites that displayed a bi-directional change on elimination or hard-wiring of auto-editing. Finally,eagsite 7 (eag7) is a novel RNA editing site that only appears on elimination of auto-editing. (d) Diagrammatic representation of three distinct neuronal subtypes: a neuron in whichdAdarauto-editing is lacking (S), a neuron in which edited and unedited states ofdAdarare present at wild-type levels (LoxP), and a neuron in whichdAdarauto-editing is at maximum (G).dAdarauto-editing regulates the editing levels of the four adenosines in a site-specific manner. While the levels of editing ofshaker site 3 are the same between the three different neuronal subtypes,ardsite 3 andunc-13site 1 exhibit differential editing levels depending on the degree ofdAdarauto-editing. Finally,eagsite 7 is only edited in neurons where auto-editing is absent, or possibly very low. Figure 8: Environmental modulation of dADAR auto-editing. ( a–b ) Auto-editing levels in adult males kept at differing temperatures for 72 h. Representative electropherograms are shown in ( a ), and averaged data in ( b ). Experimental temperatures are indicated. n =3 RT–PCRs per population. **: P <0.005, ***: P <0.0005, one-way ANOVA with Dunnett post-hoc test. Error bars, s.e.m. ( c ) Model depicting the functional consequences of neuron-to-neuron variation in auto-editing. The graph depicts the change in editing of four substrate adenosines in the dAdar WTLoxP , dAdar S , and dAdar G genetic backgrounds. Shaker site 3 (sha3) belongs to the category of editing sites that was insensitive to the edited status of dAdar . Unc-13 site 1 (unc1) belongs to the class of editing sites that displayed no effect on elimination of auto-editing, but exhibited a significant reduction on hard-wiring of dAdar auto-editing, whereas ard site 3 (ard3) belongs to the group of editing sites that displayed a bi-directional change on elimination or hard-wiring of auto-editing. Finally, eag site 7 (eag7) is a novel RNA editing site that only appears on elimination of auto-editing. ( d ) Diagrammatic representation of three distinct neuronal subtypes: a neuron in which dAdar auto-editing is lacking (S), a neuron in which edited and unedited states of dAdar are present at wild-type levels (LoxP), and a neuron in which dAdar auto-editing is at maximum (G). dAdar auto-editing regulates the editing levels of the four adenosines in a site-specific manner. While the levels of editing of shake r site 3 are the same between the three different neuronal subtypes, ard site 3 and unc-13 site 1 exhibit differential editing levels depending on the degree of dAdar auto-editing. Finally, eag site 7 is only edited in neurons where auto-editing is absent, or possibly very low. Full size image Drosophila ADAR and mouse ADAR2 primarily contribute to nervous system function through their ability to diversify the neuronal proteome via mRNA re-coding [5] , [8] . Intriguingly, both of these ADAR homologues have evolved auto-regulatory feedback loops as a mechanism to optimize enzyme function [22] , [23] , [24] . Here we have used ends-out homologous recombination to define the role of dAdar auto-editing at the molecular, cellular and behavioural levels. Although in vitro data have suggested that auto-editing might broadly reduce enzymatic function on all substrates [22] , our data demonstrates that, in vivo , only a fraction of Drosophila RNA-editing sites are modulated by dAdar auto-regulation. Furthermore, this modulation is distinctly non-uniform, with adenosines showing either mono- or bi-directional alterations in the degree of editing on hard-wiring or abolishing dAdar auto-editing. Thus, post-transcriptional auto-regulation of dADAR activity induces a complex alteration in the magnitude of deamination across the spectrum of edited adenosines, adding a further multi-faceted regulatory layer to control mRNA re-coding, in addition to spatio-temporal regulation of dADAR expression and alternative splicing [23] . How does such a non-uniform response arise? A comparison of reductions in editing in dAdar G hemizygotes and those in a recently engineered hypomorphic allele of dAdar ( dAdar hyp ) indicates that auto-editing effectively acts to generate a weakly hypomorphic allele of dAdar , rather than to modify substrate-specificity. Importantly, we provide a mechanistic basis for such an effect: the sequestration of auto-edited dADAR proteins to an, as yet unidentified, nuclear sub-compartment, thus potentially lowering the active concentration of dADAR at sites of transcription. In mammalian cells, transcripts with high inosine content are often retained within the nucleus in paraspeckle-associated complexes [32] , [33] , [34] . We speculate that auto-edited dADAR specifically binds to a similar dsRNA source within paraspeckle-like domains in Drosophila neurons. It should also be noted, however, that auto-editing still affects catalytic function even in an in vitro system [22] . Thus, we cannot rule out the possibility that alterations in dADAR catalysis, through auto-editing, also contributes to the results observed in vivo . Both sequestration of dADAR and a reduction in the efficiency of substrate deamination may act synergistically to define the net effect of auto-editing. Our findings suggest an intriguing convergent function of dADAR and mammalian ADAR2 auto-editing. De novo generation of an AI splicing acceptor site by ADAR2, in its own transcript, results in a frame-shift that forces the translational machinery to initiate from an internal methionine at lower efficiency, thus reducing ADAR2 protein levels [24] . Our data indicates that Drosophila deploys a distinct molecular strategy to achieve a similar regulatory outcome: dAdar auto-editing does not reduce the total levels of dADAR, but instead acts to alter catalysis and limit the concentration of dADAR at active sites of transcription. One surprising discrepancy between our in vivo data and previous in vitro experiments is the effect of auto-editing on deamination of dADAR's own transcript. In vitro , dAdar mRNA is robustly edited by the genomically encoded dADAR, but only weakly by its auto-edited counterpart [22] . This differential feedback would be expected to result in total auto-editing levels within a given neuron reaching an equilibrium value that would exhibit minimal variability between different neurons. Regional differences in dADAR expression would be unlikely to result in substantial deviation from this equilibrium, because large reductions in dADAR levels do not strongly affect auto-editing levels [28] . However, we found no evidence for such feedback in vivo , suggesting that dAdar auto-editing could be controlled in a cell-specific manner. Supporting this concept, we found sex-specific regulation of auto-editing in the adult thorax and species-specific divergences in spatial patterns of auto-editing. Using a novel in vivo fluorescent reporter of dADAR activity, we have recently shown that auto-editing is also differentially regulated within distinct neuronal sub-populations in the Drosophila brain [35] . In concert with the findings presented in this paper detailing the molecular consequences of dADAR auto-editing, our data suggests that auto-editing levels are set on a neuron-to-neuron basis and may contribute to the optimization of cellular physiology by generating cell-specific repertoires of differentially modified ion channels and synaptic release proteins ( Fig. 8c,d ). In concordance with this hypothesis, we observed alterations in adult behaviour in males containing dAdar alleles either abolishing or hard-wiring auto-editing. Interestingly, the behavioural defects observed in dAdar G males (such as reduced locomotor activity and an increase in the latency to court females) are also observed to a greater degree in dAdar hypomorphs [28] , in agreement with the concept that the effect of auto-editing phenocopies a weak hypomorphic variant of dADAR. The mechanistic basis for spatial regulation of auto-editing is unknown. One attractive hypothesis is that the degree of auto-editing is controlled by trans -acting factors whose expression varies between tissues (and potentially between neurons), thus explaining the discrepancy between our in vivo data and dADAR's actions in vitro [22] . Our data has also uncovered an unexpected abiotic regulation of dADAR auto-editing. Reducing or increasing the external temperature for a relatively short period (72 h) induced significant shifts in the magnitude of dADAR auto-editing, presumably as a combinatorial consequence of altered dADAR catalysis and temperature-induced changes in the structural stability of the substrate within the dAdar transcript. It will be intriguing to examine the effect of temperature-changes on the remainder of the Drosophila editing sites, and whether the temperature-induced modifications in dADAR auto-editing act to buffer or enhance any alterations in other dADAR targets. If this phenomenon is broadly applicable, environmental fluctuations in temperature have the capacity to substantially and specifically modify the proteomic content of the nervous systems of insect and other poikilothermic species via altered RNA editing. In summary, our results greatly expand on previous methods used to investigate dAdar auto-regulation and yield distinct paradigms in relation to the functional consequences of dAdar auto-editing in an in vivo setting. These findings further elaborate the complex nature of A-to-I RNA editing in the Drosophila nervous system and the multi-layered regulatory mechanisms that control mRNA re-coding, neuronal physiology and behaviour. Drosophila stocks and homologous recombination Drosophila were raised at a constant 25 °C, on standard molasses food and under 12-h day/night cycles. For analysis of RNA editing, RNA was derived from 3- to 5-day-old flies. For experiments involving dAdar null males, we used the dAdar 5g1 allele, previously shown to lack all detectable RNA-editing activity [6] . Stocks of D. simulans , D. sechellia , D. yakuba and D. erecta were obtained from the Drosophila Species Stock Center (University of California, San Diego). Extensive details of the constructs used to manipulate the dAdar locus, using homologous recombination, have been published previously [28] . Briefly, we cloned two arms encompassing exons 4–7 (arm 1) and 8–10 (arm 2) of the dAdar genomic sequence into the p[w25.2] vector. We used mutagenic primers to convert the endogenous AGT serine codon to a synonymous TCT codon or a GGT glycine codon. An arm 1 with an AGT codon served as a control. Arm 2 contains a HA epitope-tag immediately after the last coding amino acid of dADAR, and before an opal (TGA) stop codon. Following recombination, the white + mini-gene selection cassette was removed via cre-recombinase and each recombinant strain was back-crossed into a Canton-S control stock for at least five generations. PCR and computational calculation of editing levels RNA extractions from Drosophila tissues were performed using TRIzol (Invitrogen). Edited cDNAs were amplified via RT–PCR using target-specific primers ( Supplementary Table S2 ). To computationally calculate editing ratios of the chosen 100 editing sites, edited adenosines were initially selected from RT–PCR electropherograms via an automated search for the local sequence surrounding the edited adenosine. All sequential peaks were then fit with a Gaussian mixture model ( Supplementary Fig. S8a ). This prevents errors in which neighbouring peaks of the same nucleotide artificially inflate the area under the curve. A grid search determines the relative positions of the peaks, and a Markov Chain Monte Carlo process is used to find the best values for height (h), width (w), and standard deviation (c), as determined by the minimum χ 2 of the sum of the areas of the predicted peaks and the chromatogram data ( Supplementary Fig. S8b ). A minimum of three independent PCR amplicons were used to derive the editing levels for each adenosine. To determine the degree of auto-editing in male hemizygotes and females heterozygous for various engineered dAdar alleles, we used the following methodology: dAdar S and dAdar G males and females were assumed to have auto-editing levels of 0% and 100%. respectively. For the remaining genotypes, auto-editing was calculated using bulk RT–PCR electropherograms of the dAdar mRNA from male and female heads, with the per cent auto-editing calculated as G/(A+G)×100. For dAdar S / dAdar WTLoxP females, harbouring both TCT and AGT serine alleles, the total level of un-edited dAdar was calculated by summating the A and T peaks. The auto-editing level was then derived as G/(A+T+G)×100. Confocal microscopy and western blotting All confocal images were obtained on a Zeiss LSM 510 meta confocal microscope. Adult brain and 3rd instar larval salivary glands were fixed in 4% PFA and blocked in 5% normal goat serum before antibody incubation. Primary antibodies were used at the following concentrations: rabbit anti-HA (Santa Cruz Biotech), 1:50; goat anti-human fibrillarin (kind gift of K.M.Pollard, TSRI, San Diego, CA), 1: 200; mouse anti-Lamin (Developmental Studies Hybridoma Bank), 1:40; 4,6-diamidino-2-phenylindole (DAPI) (Invitrogen) was used at 1:1,000. Images were contrast-enhanced in Adobe Photoshop. Protein samples were prepared in buffer containing SDS and β-mercaptoethanol, and run out on a 10% gel (Amresco). Anti-HA antibody (Covance) was used at 1:500, and anti-actin (Millipore) was used at 1:20,000. Band intensities were quantified on a Kodak Image Station following background subtraction. 20 adult heads per 100 μl of buffer were used per sample. To quantify the degree of extranucleolar punctal dADAR, images were split by hand into individual cells, using DAPI as a marker for nuclear location (blue). For each cell, the nucleolus, N, is defined as the contiguous region surrounding the brightest pixel of fibrillarin staining (red), F, where the intensity of every pixel is greater than 1/4 of F. The region of dADAR staining (green), P, was similarly identified. P is defined as the contiguous region surrounding the brightest pixel of dADAR staining, A, where the intensity of every pixel is greater than 1/2 of A. For the measures P/D and # P >0, which examine extra-nucleolar punctate dADAR staining, P is considered 0, unless it is punctate (the area of P is less than the area of N) and extranucleolar (the position of A lies outside the area of N) ( Supplementary Fig. S4 ). Behavioural analysis Locomotor patterns were recorded using horizontal single fly or vertical population activity monitors (TriKinetics). For single-fly monitors, mean locomotor patterns were calculated for each fly by averaging data from 3 consecutive days, which were then further averaged across the experimental population. To quantify climbing ability using vertical population monitors, we took advantage of the presence of three concentric infra-red beams at the bottom, middle and top portions of the vial. We calculated the total number of beam breaks for all levels, and solely for the top level (close to the top of the vial). Relative climbing ability was calculated by dividing the number of beams breaks in the top ring by the total for all three rings, for each vial. Analysis of circadian parameters (period, per cent rhythmicity and power) was performed using FaasX (M. Boudinot and F. Rouyer). To analyse courtship behaviour, we measured two parameters: the time taken to initiate courtship (defined as the first orientation of the male to the female), and the total time spent courting. Males were aged for 5–7 days, and female virgins 3–5 days, before single-fly pairing. We used a custom-made chamber to observe behaviour. Courtship occurs in circular chamber with a diameter of ~1 cm and height ~0.5 cm. To recapitulate ethologically relevant conditions, live, rather than decapitated, females were used. To control for circadian influences on behaviour, experiments were performed in a relatively narrow time window (8–11 am). Attempted mating was observed over a 10 min time-span, or until the male successfully copulated. How to cite this article: Savva, Y. A. et al . Auto-regulatory RNA editing fine-tunes mRNA re-coding and complex behaviour in Drosophila . Nat. Commun. 3:790 doi: 10.1038/ncomms1789 (2012).